Cortical representations of confidence in a visual perceptual decision To date the exact neuronal implementation of decision confidence has been subject to little research. Here we explore electroencephalographic correlates of human choice certainty in a visual motion discrimination task for either spatial attention or motor effector cue instructions. We demonstrate electrophysiological correlates of choice certainty that evolve as early as 300 ms after stimulus onset and resemble the primary visual motion representations in early visual cortex. These correlates do not emerge unless or until the subject unambiguously knows which of the competing visual stimuli is actually relevant to behaviour. They extend beyond stimulus presentation up to the motor response but are independent of the motor effector. Our findings suggest that perceptual confidence evolves in parallel with representations of stimulus properties and is dedicated to one specific aspect of the visual world. Its electroencephalographic correlates can be disentangled from representations of sensory evidence, objective discrimination performance and overt motor behaviour. Natural perceptual systems have to cope with systematic uncertainty as sensory information is noisy and insufficient to uniquely determine the environment. Accordingly, visual perception has been described as a process of inference by which ambiguous sensory cues are combined with internal knowledge of the world to arrive at a consistent interpretation of the scene [1] , [2] . The Bayesian statistical theory frames this problem quantitatively and has been successfully applied to cognitive phenomena in perception [3] , [4] and sensorimotor learning [5] , [6] . To optimize behaviour as per the Bayes’ rule, subjective certainties reflecting non-dichotomous conditional probabilities [7] of both previous knowledge and sensory input determine their optimal weighting in every perceptual decision. Neuronal recordings in behaving monkeys [7] , [8] and rats [9] have detected representations of decision formation and the degree of certainty in it. For perceptual decisions—such as a monkey’s discrimination of visual motion direction in a noisy random dot display and reporting it by an eye movement—neural correlates have been demonstrated in a sensorimotor association area that is concerned with the preparation of the actions. When monkeys report the perceived direction of visual motion by a saccadic eye movement, lateral intraparietal cortex (LIP) neurons represent the accumulation of evidence [8] as well as choice certainty [7] . This pool of neurons gradually increases or decreases its firing rate as more evidence mounts for or against one of the choices; LIP neurons sustain a discharge that determines the outcome of the decision when the accumulated evidence reaches a critical level. The exact neurobiology underlying the negotiation of this threshold and the underlying evidence is not currently known. Yet theoretical and experimental data suggest that the neural computations approximate a form of probabilistic reasoning featuring choice certainty [3] , [7] , [10] . Surprisingly, to date there is little electrophysiological evidence on human choice certainty [11] . In a recent psychophysical study, we investigated the influence of spatial and feature-based attention on human choice certainty using a motion discrimination task and a certainty wager similar to a pioneering experiment in behaving monkeys [7] . Complemented by numerical confidence ratings, our data revealed a dissociation of choice accuracy and certainty with a significantly stronger influence of voluntary top-down attention on subjective performance measures than on objective performance [12] . Selective attention is capable of dissociating a perceptual decision and the confidence in it by affecting them differently. In the electroencephalographic (EEG) experiments presented here, we sought to characterize the electrophysiological signatures of human choice certainty and further clarify the role of this metacognitive evaluation in motor preparation. Since in non-human primates choice certainty is encoded by the same population of neurons as the perceptual decision and the saccadic eye movement indicating the direction decision [7] , [8] , we here separated perceptual integration and motor planning by requesting subjects to report their decision by hand movements in delayed-response paradigms. To dissociate physiological representations of objective performance and subjective confidence even further, in a first experiment we asked one group of subjects to indicate the perceived direction of moving random dots and the confidence in that perceptual decision while stimuli were cued validly and invalidly [12] , [13] , [14] . In the second experiment, we did not cue selective attention but the motor effector to identify electrophysiological correlates of decision confidence in motor preparation. Our findings suggest that perceptual confidence evolves in parallel with representations of stimulus properties and is dedicated to specific aspects of visual stimuli. Experiment 1 While 30-channel EEG was recorded, in the first experiment we let human subjects discriminate global visual motion embedded in noise for validly and invalidly cued stimuli ( Fig. 1a ) and rate the confidence in their perceptual decision. Both four-alternative forced choice responses were acquired trial by trial. Subjects observed two random dot kinematograms (RDKs) presented simultaneously in their left and right visual hemifield. While a precue indicated which RDK to attend to with 80% validity, participants did not know definitely which one of the two would prove behaviourally relevant until postcue onset following stimulus presentation. Subjects indicated the direction of perceived global visual motion using their right hand via a first button press (up, down, left or right), by the following button press they rated their confidence on a scale of 0–3 ( 0 being ‘I guessed’, 3 ‘I was sure’). 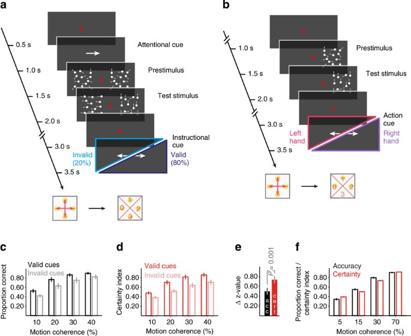Figure 1: Task design and behavioural data for Experiment 1 and 2. (a) Experiment 1: timing of events for an example trial: the test stimulus consisted of two random dot kinematograms (RDKs) presented simultaneously left and right of the fixation point (1.5–2 s), level of motion coherence and direction of global motion (four alternatives) was modulated on a trial-by-trial basis. An arrow before stimulus presentation (0.5–1 s) indicated which RDK covertly shift attention to, a second arrow after the stimulus (3–3.5 s) instructed subjects which RDK they actually had to report the direction of coherent motion for. Valid cueing of spatial selective attention—as defined by congruent orientation of the attentional and the instructional cue—was applied in 80% of trials, see dark blue option. Invalid cueing (incongruent arrows, light blue option) was applied in the remaining 20% of trials. Subjects reported perceived motion direction with a first button press and decision certainty with either a second press of the same buttons using four predefined numerical ratings. (b) Experiment 2: this slight variation involved no cueing of selective attention, but an instruction as to which hand to respond with. Timing of events corresponded toa, but the attentional cue (0.5–1 s) was substituted by an extended fixation period. Prestimulus and test stimulus were randomly presented in the left or right visual hemifield, and instead of the postcue (3–3.5 s) an action cue was presented instructing subjects randomly as to which hand to respond with. (c) Experiment 1, proportion of correct responses for the four motion coherence levels and the two cueing conditions separately, all subjects. (d) Experiment 1, certainty index for the four motion coherence levels and the two cueing conditions separately, all subjects. (e) Experiment 1, selective attention increased both z-standardized proportion of correct responses (accuracy) and certainty as indicated by positive z-values, all subjects. Certainty increased significantly more with attention than accuracy (t-test:P=0.001). (f) Experiment 2, proportion of correct responses and certainty index for the four motion coherence levels, all subjects. All bar charts display mean±s.e.m. Figure 1: Task design and behavioural data for Experiment 1 and 2. ( a ) Experiment 1: timing of events for an example trial: the test stimulus consisted of two random dot kinematograms (RDKs) presented simultaneously left and right of the fixation point (1.5–2 s), level of motion coherence and direction of global motion (four alternatives) was modulated on a trial-by-trial basis. An arrow before stimulus presentation (0.5–1 s) indicated which RDK covertly shift attention to, a second arrow after the stimulus (3–3.5 s) instructed subjects which RDK they actually had to report the direction of coherent motion for. Valid cueing of spatial selective attention—as defined by congruent orientation of the attentional and the instructional cue—was applied in 80% of trials, see dark blue option. Invalid cueing (incongruent arrows, light blue option) was applied in the remaining 20% of trials. Subjects reported perceived motion direction with a first button press and decision certainty with either a second press of the same buttons using four predefined numerical ratings. ( b ) Experiment 2: this slight variation involved no cueing of selective attention, but an instruction as to which hand to respond with. Timing of events corresponded to a , but the attentional cue (0.5–1 s) was substituted by an extended fixation period. Prestimulus and test stimulus were randomly presented in the left or right visual hemifield, and instead of the postcue (3–3.5 s) an action cue was presented instructing subjects randomly as to which hand to respond with. ( c ) Experiment 1, proportion of correct responses for the four motion coherence levels and the two cueing conditions separately, all subjects. ( d ) Experiment 1, certainty index for the four motion coherence levels and the two cueing conditions separately, all subjects. ( e ) Experiment 1, selective attention increased both z-standardized proportion of correct responses (accuracy) and certainty as indicated by positive z-values, all subjects. Certainty increased significantly more with attention than accuracy ( t -test: P =0.001). ( f ) Experiment 2, proportion of correct responses and certainty index for the four motion coherence levels, all subjects. All bar charts display mean±s.e.m. Full size image Objective and subjective performance measures Reflecting the dependency of task difficulty on motion coherence, discrimination performance increased for higher motion coherences in both attention conditions as expected [12] , [14] . Furthermore, we found higher sensitivity to visual motion for valid as compared with invalid cues as indicated by higher mean accuracy with attention for each of the four coherence levels (mean accuracy for 10/20/30/40% coherence, valid cues: 0.53/0.77/0.87/0.90; invalid cues: 0.42/0.63/0.75/0.83; Fig. 1c ). That is, for a given coherence level attention increased the proportion of correct choices. This improvement in performance for an attended stimulus is the signature of attentional modulation on behaviour [15] and demonstrates that subjects reliably followed the cue instructions. Decision confidence—as expressed by a certainty index (see Methods for details)—varied with cueing conditions, as well: post-decision certainty for valid cue trials was significantly higher than for invalid cue trials (mean certainty index: 0.62 versus 0.41; t -test: P <0.001), certainty indices for valid and invalid cues differed significantly for all four coherence levels ( t -tests for all contrasts: P ≤0.001). Similar to the effect in objective performance, certainty indices increased with higher motion coherence (mean certainty index for 10/20/30/40% coherence, valid cues: 0.48/0.71/0.82/0.86; invalid cues: 0.39/0.52/0.64/0.71; Fig. 1d ). There was a significant difference between certainty indices of all four coherence levels for valid and invalid cues separately ( t -test for all contrasts: P ≤0.001). Accordingly, mean motion coherence underlying the highest certainty ratings was significantly higher than mean motion coherence underlying the lowest certainty ratings for both cueing conditions (valid cues: 30.9% versus 17.1%, t -test: P <0.001; invalid cues: 31.8% versus 19.2%, t -test: P <0.001). Increases of mean confidence with attention were more pronounced than for choice accuracy. This indicates an even stronger effect of selective attention on post-decision certainty as compared with choice accuracy. To quantify and further investigate this attention-related variation, every subject’s mean accuracy and certainty of the four coherence levels each for valid and invalid cues were z-transformed to a common mean (0) and s.d. (1). In accordance with our previous study [12] , paired t -tests on these standardized measures revealed not only significant increases for decision accuracy and choice confidence with attention (both t -tests: P <0.001; Fig. 1e , positive Δ z-values for each category), but also a significantly stronger increase of the confidence measure ( t -test: P =0.001; labelled grey in Fig. 1e ). Similarly, response times (RTs) varied with stimulus properties. Following the offset of the second arrow (3.5 s), subjects would indicate the direction of coherent motion and their choice certainty. RTs were significantly faster in valid cue trials (valid: mean=4.033±0.139 s; invalid: mean=4.358±0.180 s; t -test: P <0.001). Both in valid and invalid cue trials, responses were significantly faster for correct motion discrimination (valid: mean correct=4.000±0.125 s, mean incorrect=4.146±0.168 s; t -test: P <0.001; invalid: mean correct=4.299±0.179 s, mean incorrect=4.536±0.290 s; t -test: P <0.024). Subjects were faster to respond to higher coherence levels with a significant difference of highest and lowest coherence for valid cues (valid: mean for 40% coherence=4.008±0.152 s, mean 10%=4.063±0.140 s; t -test: P =0.036; invalid: mean 40%=4.323±0.234 s, mean 10%=4.416±0.216 s; t -test: P =0.280). RTs were faster with higher choice certainty with significant differences between highest and lowest confidence levels for both cueing conditions (valid: mean for certainty 3 =3.953±0.113 s, mean 0 =4.204±0.327 s; t -test: P =0.018; invalid: mean 3 =4.052±0.125 s, mean 0 =4.592±0.342 s; t -test: P <0.001). 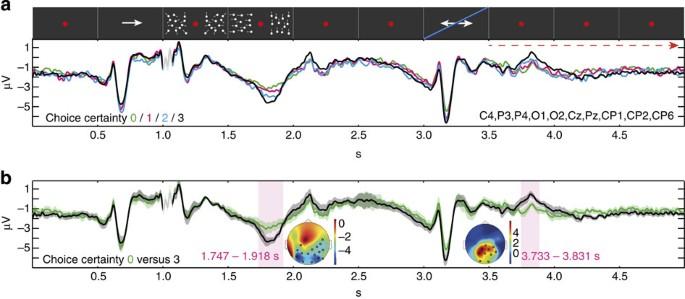Figure 2: Differences between confidence ratings in Experiment 1. (a) Symbolic representation of the visual stimulus along the stimulus-locked grand-average event-related potential (ERP) responses. Different colours represent ERPs for the four different confidence ratings, on a scale of 0–3 (from0being ‘I guessed’, to3‘I was sure’). (b) Stimulus-locked grand-average ERP responses to highest versus lowest confidence ratings differed in two time intervals (indicated by pink areas). Headplots of the nonparametric cluster-randomization approach (two-tailedt-test, corrected for multiple comparisons at a cluster-level,P<0.050) map the scalp distribution of statistical differences of ‘I was sure’ versus ‘I guessed’ ratings from 1.747 to 1.918 s (negative cluster;P=0.001) and from 3.733 to 3.831 s (positive cluster;P<0.001). Heat colours of the maps represent thet-values of the statistical comparisons (colour bar indicatest-values, relative scaling is specific to each topoplot) and the black circles represent electrodes that contribute to the significant cluster. ERP responses are averages over all electrodes that were part of the late significant cluster and are plotted with s.e. values of the mean inb(shaded areas). The ERP discontinuity around 1.0 s indicates an artefact due to the synchronization pulse of EEG and presentation computer. Electrophysiological correlates of decision confidence Figure 2a superimposes the grand-average event-related potentials (ERPs) of the subjects’ four certainty levels time-locked to the onset of the trials. A schematic of the behavioural task sequence is displayed along with the course of the ERP. Following the appearance of the precue at 0.5 s and postcue arrow at 3.0 s as well as following RDK onset at 1.0 s and offset at 2.0 s, we observed distinctive visual-evoked potentials. In that all EEG electrodes were referenced to FCz, the first prominent deflection after each of these four points in time at about 120 ms conformed to common visual N100 effects, the second at about 225 ms to P200 effects. A further peak observed at around 300 ms after the postcue was identified to represent a classical P300 effect (see for example, polarity of ERP components in exemplary grand-average ERPs for valid and invalid trials referenced to linked mastoids in Fig. 3 ). Averaged across certainty ratings, ERPs revealed two pronounced dissociations of brain electrical activity that differed in polarity and localization. With increasing post-decision certainty, we observed monotonically increasing negative potential shifts during the presentation of the test stimulus (1.5 to 2.0 s) and ascendingly positive potential shifts about 300–400 ms after the onset of the response window at 3.5 s (red arrow in Fig. 2a ). In a statistical comparison of lowest and highest certainty trials ( Fig. 2b ), these components were expressed by a significant negative cluster ( P =0.001) over parieto-occipital electrodes that was present from 1.747 to 1.918 s and a large, significant positive cluster ( P <0.001) from 3.733 to 3.831 s. Figure 2: Differences between confidence ratings in Experiment 1. ( a ) Symbolic representation of the visual stimulus along the stimulus-locked grand-average event-related potential (ERP) responses. Different colours represent ERPs for the four different confidence ratings, on a scale of 0–3 (from 0 being ‘I guessed’, to 3 ‘I was sure’). ( b ) Stimulus-locked grand-average ERP responses to highest versus lowest confidence ratings differed in two time intervals (indicated by pink areas). Headplots of the nonparametric cluster-randomization approach (two-tailed t -test, corrected for multiple comparisons at a cluster-level, P <0.050) map the scalp distribution of statistical differences of ‘I was sure’ versus ‘I guessed’ ratings from 1.747 to 1.918 s (negative cluster; P =0.001) and from 3.733 to 3.831 s (positive cluster; P <0.001). Heat colours of the maps represent the t -values of the statistical comparisons (colour bar indicates t -values, relative scaling is specific to each topoplot) and the black circles represent electrodes that contribute to the significant cluster. ERP responses are averages over all electrodes that were part of the late significant cluster and are plotted with s.e. values of the mean in b (shaded areas). The ERP discontinuity around 1.0 s indicates an artefact due to the synchronization pulse of EEG and presentation computer. 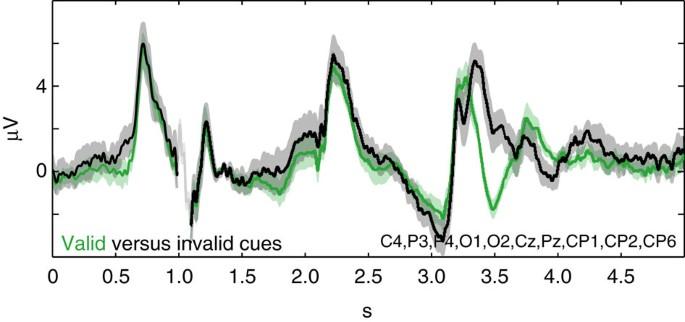Figure 3: Linked-mastoid grand-average ERP responses to valid cue and invalid cue trials in Experiment 1. Valid cues were presented in 80% of the trials, hence for the infrequent invalid cues about 300 ms after the postcue (postcue start time: 3.0 s) a classical P300 component was observed. ERP responses are averages over electrodes C4, P3, P4, O1, O2, Cz, Pz, CP1, CP2, CP6 and are plotted with s.e. values of the mean (shaded areas). The ERP discontinuity around 1.0 s indicates an artefact due to the synchronization pulse of EEG and presentation computer. Full size image Figure 3: Linked-mastoid grand-average ERP responses to valid cue and invalid cue trials in Experiment 1. Valid cues were presented in 80% of the trials, hence for the infrequent invalid cues about 300 ms after the postcue (postcue start time: 3.0 s) a classical P300 component was observed. ERP responses are averages over electrodes C4, P3, P4, O1, O2, Cz, Pz, CP1, CP2, CP6 and are plotted with s.e. values of the mean (shaded areas). The ERP discontinuity around 1.0 s indicates an artefact due to the synchronization pulse of EEG and presentation computer. Full size image Do factors that covary with confidence—like motion coherence and attention—contribute to the effects seen here? First, choice certainty was inspected for valid and invalid cue trials separately. As stimuli were not varied systematically until the test stimulus started, the following ERPs are plotted starting at around 1.5 s. Contrasting the four confidence ERPs of valid cues ( Fig. 4a ) with the respective ERPs of invalid cues ( Fig. 4b ), the early dissociation during test stimulus presentation persisted for both cueing conditions. For highest versus lowest certainty, this difference was expressed by a significant negative cluster from 1.742 to 1.931 s in valid ( P =0.001; Fig. 4e ) and from 1.765 to 1.870 s in invalid cue trials ( P =0.005; Fig. 4g ). The second significant dissociation seen in the pooled data above, however, was observed for valid cue trials only. It was expressed by a significant positive cluster ( P =0.024) of parieto-occipital electrodes ( Fig. 4f ) that was present from 3.742 to 3.823 s. By analysing the ERPs for the two cueing conditions separately, the influence of invalid cueing could be determined as well. As expected, visual inspection showed nearly congruent waveforms up to the presentation of the second arrow defining the cueing condition at 3.0 s. Two negative shifts peaking at about 200 and 350 ms, respectively, after the postcue were observed, the second one for invalid cue trials only. We consider the first deflection to be a P200 component as mentioned above, the second for the 20% of all trials with incongruent postcues a classical P300 component. For invalid cue trials, P200 amplitude significantly increased with choice certainty as expressed by a large negative cluster ( P =0.003) that was present from 3.146 to 3.263 s and was pronounced over the right hemisphere ( Fig. 4h ). In distribution and polarity, this increase very much resembled the one observed for the dissociation of certainty ERPs during test stimulus presentation in both valid and invalid cue trials (see for example, Fig. 4e,g ). The difference between the highest and lowest certainty ratings just missed significance for the P300 component. 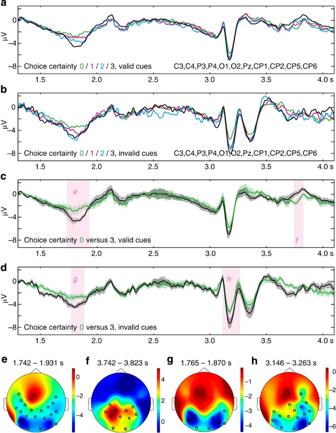Figure 4: Differences between confidence ratings in Experiment 1 for valid cue and invalid cue trials. (a,b) Stimulus-locked grand-average certainty ERP responses to valid cue (a) and invalid cue trials (b). Different colours represent ERPs for the four different confidence ratings, on a scale of 0–3 (from0being ‘I guessed’, to3‘I was sure’). (c,d) Stimulus-locked grand-average ERP responses to highest versus lowest confidence ratings in valid cue (c) and invalid cue trials (d) differed in four time intervals (indicated by pink areas). (e–h) Headplots of the nonparametric cluster-randomization approach (two-tailedt-test, corrected for multiple comparisons at a cluster-level,P<0.050) map the scalp distribution of statistical differences of ‘I was sure’ versus ‘I guessed’ ratings. Heat colours of the maps represent thet-values of the statistical comparisons (colour bar indicatest-values, relative scaling is specific to each topoplot) and the black circles represent electrodes that contribute to the significant cluster. (e) Negative cluster from 1.742 to 1.931 s in valid cue trials (P=0.001). (f) Positive cluster from 3.742 to 3.823 s in valid cue trials (P=0.024). (g) Negative cluster from 1.765 to 1.870 s in invalid cue trials (P=0.005). (h) Negative cluster from 3.146 to 3.263 s in invalid cue trials (P=0.003). ERP responses are averages over all electrodes that were part of the late significant cluster in valid cue trials (f) and are plotted with standard errors of the mean inc,d(shaded areas). Figure 4: Differences between confidence ratings in Experiment 1 for valid cue and invalid cue trials. ( a , b ) Stimulus-locked grand-average certainty ERP responses to valid cue ( a ) and invalid cue trials ( b ). Different colours represent ERPs for the four different confidence ratings, on a scale of 0–3 (from 0 being ‘I guessed’, to 3 ‘I was sure’). ( c , d ) Stimulus-locked grand-average ERP responses to highest versus lowest confidence ratings in valid cue ( c ) and invalid cue trials ( d ) differed in four time intervals (indicated by pink areas). ( e – h ) Headplots of the nonparametric cluster-randomization approach (two-tailed t -test, corrected for multiple comparisons at a cluster-level, P <0.050) map the scalp distribution of statistical differences of ‘I was sure’ versus ‘I guessed’ ratings. Heat colours of the maps represent the t -values of the statistical comparisons (colour bar indicates t -values, relative scaling is specific to each topoplot) and the black circles represent electrodes that contribute to the significant cluster. ( e ) Negative cluster from 1.742 to 1.931 s in valid cue trials ( P =0.001). ( f ) Positive cluster from 3.742 to 3.823 s in valid cue trials ( P =0.024). ( g ) Negative cluster from 1.765 to 1.870 s in invalid cue trials ( P =0.005). ( h ) Negative cluster from 3.146 to 3.263 s in invalid cue trials ( P =0.003). ERP responses are averages over all electrodes that were part of the late significant cluster in valid cue trials ( f ) and are plotted with standard errors of the mean in c , d (shaded areas). Full size image Mean motion coherence was higher in more certain responses: 16.96% for certainty rating 0 , 19.11% for 1 , 23.50% for 2 , 30.91% for 3 in valid and 19.21% for 0 , 23.37% for 1 , 28.12% for 2 , 31.85% for 3 in invalid cues. Therefore, ERP differences seen for the different certainty levels during test stimulus presentation could basically be explained by underlying motion coherence. To test whether differences in ERPs observed for the different certainty levels ( Figs 2 and 4 ) are secondary to differences induced by visual stimulation, we also examined the impact of the presented motion coherence on the effects observed for choice certainty and cueing conditions. 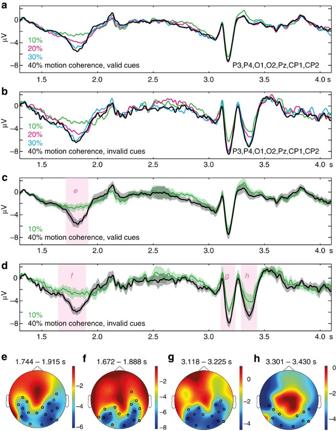Figure 5: Differences between presented motion coherence levels in Experiment 1 for valid cue and invalid cue trials. (a,b) Stimulus-locked grand-average coherence ERP responses to valid cue (a) and invalid cue trials (b). Different colours represent ERPs for the four different levels of motion coherence (10, 20, 30 and 40%) presented in the experiment. (c,d) Stimulus-locked grand-average ERP responses to the highest and the lowest coherence level in valid cue (c) and invalid cue trials (d) differed in four time intervals (indicated by pink areas). (e–h) Headplots of the nonparametric cluster-randomization approach (two-tailedt-test, corrected for multiple comparisons at a cluster-level,P<0.050) map the scalp distribution of statistical differences of 40 versus 10% motion coherence. Same conventions as inFig. 2, colour bar indicatest-values, relative scaling is specific to each topoplot. (e) Negative cluster from 1.744 to 1.915 s in valid cue trials (P=0.001). (f) Negative cluster from 1.672 to 1.888 s in invalid cue trials (P<0.001). (g) Negative cluster from 3.118 to 3.225 s in invalid cue trials (P=0.008). (h) Negative cluster from 3.301 to 3.430 s in invalid cue trials (P=0.008). ERP responses are averages over electrodes P3, P4, O1, O2, Pz, CP1, CP2 and are plotted with s.e. values of the mean inc,d(shaded areas). Figure 5 side-by-side displays the ERPs for the four motion coherence levels—10, 20, 30, and 40%—presented in the experiment. For valid ( Fig. 5a ) and invalid cues alike ( Fig. 5b ), with increasing motion coherence the onset of the coherent motion signal at 1.5 s elicited monotonically increasing negative potential shifts. Cluster-level randomization tests identified a larger negative deflection over parieto-occipital electrodes for 40% motion coherence as compared with 10% coherence from 1.744 to 1.915 s in valid ( Fig. 5e ) and from 1.672 to 1.888 s in invalid trials ( Fig. 5f ). Interestingly, a similar ERP dissociation was also observed later in the course of the trial, this time for invalid cues only. For invalid as opposed to valid cues, the two prominent potential components following postcue onset at 3.0 s were coherence-dependent, as well (negative deflections between 3.0 and 3.5 s displayed in Fig. 5b ). We observed potential shifts to be in inverse proportion to the four presented motion coherences. Cluster statistics exemplarily highlighted larger negative deflections over parieto-occipital electrodes from 3.118 to 3.225 s ( P =0.008; Fig. 5g ) and from 3.301 to 3.430 s ( P =0.008; Fig. 5h ) for 40% as compared with 10% coherence. Thus, both the P200 and the P300 component varied with presented motion coherence, and this motion dependence for invalid cues was similar in polarity and distribution to the earlier response seen during the presentation of the motion stimulus for both cueing conditions. While cluster-level randomization tests identified significant differences between ERPs of different coherence levels during the ~250 ms preceding stimulus offset for valid and invalid cues alike ( Fig. 5e,f ), they did not for the time interval of the late certainty dissociation. This finding suggested that the early certainty correlate possibly is confounded by stimulus characteristics, the late dissociation with decision confidence, by contrast, is not. Figure 5: Differences between presented motion coherence levels in Experiment 1 for valid cue and invalid cue trials. ( a , b ) Stimulus-locked grand-average coherence ERP responses to valid cue ( a ) and invalid cue trials ( b ). Different colours represent ERPs for the four different levels of motion coherence (10, 20, 30 and 40%) presented in the experiment. ( c , d ) Stimulus-locked grand-average ERP responses to the highest and the lowest coherence level in valid cue ( c ) and invalid cue trials ( d ) differed in four time intervals (indicated by pink areas). ( e – h ) Headplots of the nonparametric cluster-randomization approach (two-tailed t -test, corrected for multiple comparisons at a cluster-level, P <0.050) map the scalp distribution of statistical differences of 40 versus 10% motion coherence. Same conventions as in Fig. 2 , colour bar indicates t -values, relative scaling is specific to each topoplot. ( e ) Negative cluster from 1.744 to 1.915 s in valid cue trials ( P =0.001). ( f ) Negative cluster from 1.672 to 1.888 s in invalid cue trials ( P <0.001). ( g ) Negative cluster from 3.118 to 3.225 s in invalid cue trials ( P =0.008). ( h ) Negative cluster from 3.301 to 3.430 s in invalid cue trials ( P =0.008). ERP responses are averages over electrodes P3, P4, O1, O2, Pz, CP1, CP2 and are plotted with s.e. values of the mean in c , d (shaded areas). Full size image To further substantiate our conclusions, we examined grand-average ERPs of highest versus lowest confidence ratings in valid cue trials for correct answers ( Fig. 6a ), for a single coherence level only (30% motion coherence; Fig. 6b ) and for the overlap of these two selections of trials ( Fig. 6c ). The late, significant dissociation seen in the pooled data above was observed similarly for all three additional analyses. Each dissociation was expressed by a significant positive cluster of parieto-occipital electrodes with similar temporal characteristics (see for example, Fig. 6d–f versus Fig. 4f). These variations of a late, significant ERP difference were observed over left-parietal electrodes and preceded the mean response time for the highest and lowest certainty level (4.079 s, valid cues only) by about 300 ms. As all subjects responded with their right hand, this finding suggested an association with the motor response. With a significant difference between response times for highest and lowest certainty in valid cues (mean RT for highest certainty 3.953 s versus lowest 4.204 s; t -test: P =0.018), in the final step of this analysis we examined motor preparation more closely. 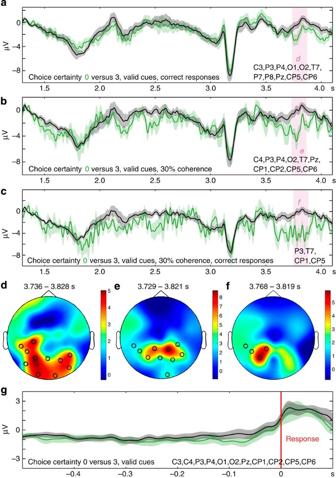Figure 6: Certainty correlates for Experiment 1. (a–c) Stimulus-locked grand-average ERP responses to highest versus lowest confidence ratings in valid cue trials: (a) for correct responses only, (b) for a single level of presented motion coherence (30% of coherently moving dots in both test stimulus dotfields), (c) for correct responses in 30% motion coherence trials. Please note that with more restrictive selection criteria fromatocthe size of the respective pool of trials decreased considerably. Each of the three ERP contrasts (a–c) differed in a similar time interval (indicated by pink areas). (d–f) Headplots of the nonparametric cluster-randomization approach (two-tailedt-test, corrected for multiple comparisons at a cluster-level,P<0.050) map the scalp distribution of statistical differences of ‘I was sure’ versus ‘I guessed’ ratings. Heat colours of the maps represent thet-values of the statistical comparisons (colour bar indicatest-values, relative scaling is specific to each topoplot) and the black circles represent electrodes that contribute to the significant cluster. (d) Positive cluster (P=0.007) from 3.736 to 3.828 s for correct responses in valid cue trials. (e) Positive cluster (P=0.002) from 3.729 to 3.821 s for 30% motion coherence in valid cue trials. (f) Positive cluster (P=0.011) from 3.768 to 3.819 s for correct responses in valid cue 30% motion coherence trials. (g) Stimulus-locked grand-average ERP responses to highest versus lowest confidence ratings in valid cue trials. Please note that both point of reference and time scaling differ from previous ERP plots as it ‘zooms’ in on the 500 ms before the discrimination response (first button press; red line). No relevant activity was detected in the averages during the time interval preceding the motor response. Cluster statistics did not reveal a significant difference between highest and lowest confidence ratings of valid cue trials for response-locked ERP responses. ERP responses are averages over all electrodes that were part of the respective significant cluster and are plotted with s.e. values of the mean (shaded areas). Figure 6g displays grand-average certainty ERPs response-locked to the first button press. ERPs did not show relevant activity for each of the two certainty levels within the 400 ms before button press. Cluster statistics did not reveal a significant difference between the two grand averages indicating that there is no certainty-specific activity time-locked to the response. Figure 6: Certainty correlates for Experiment 1. ( a – c ) Stimulus-locked grand-average ERP responses to highest versus lowest confidence ratings in valid cue trials: ( a ) for correct responses only, ( b ) for a single level of presented motion coherence (30% of coherently moving dots in both test stimulus dotfields), ( c ) for correct responses in 30% motion coherence trials. Please note that with more restrictive selection criteria from a to c the size of the respective pool of trials decreased considerably. Each of the three ERP contrasts ( a – c ) differed in a similar time interval (indicated by pink areas). ( d – f ) Headplots of the nonparametric cluster-randomization approach (two-tailed t -test, corrected for multiple comparisons at a cluster-level, P <0.050) map the scalp distribution of statistical differences of ‘I was sure’ versus ‘I guessed’ ratings. Heat colours of the maps represent the t -values of the statistical comparisons (colour bar indicates t -values, relative scaling is specific to each topoplot) and the black circles represent electrodes that contribute to the significant cluster. ( d ) Positive cluster ( P =0.007) from 3.736 to 3.828 s for correct responses in valid cue trials. ( e ) Positive cluster ( P =0.002) from 3.729 to 3.821 s for 30% motion coherence in valid cue trials. ( f ) Positive cluster ( P =0.011) from 3.768 to 3.819 s for correct responses in valid cue 30% motion coherence trials. ( g ) Stimulus-locked grand-average ERP responses to highest versus lowest confidence ratings in valid cue trials. Please note that both point of reference and time scaling differ from previous ERP plots as it ‘zooms’ in on the 500 ms before the discrimination response (first button press; red line). No relevant activity was detected in the averages during the time interval preceding the motor response. Cluster statistics did not reveal a significant difference between highest and lowest confidence ratings of valid cue trials for response-locked ERP responses. ERP responses are averages over all electrodes that were part of the respective significant cluster and are plotted with s.e. values of the mean (shaded areas). Full size image Experiment 2 In the second experiment a single RDK was presented in either the left or the right visual hemifield without selective spatial attention cueing, rather subjects were instructed as to which hand to respond with trial by trial ( Fig. 1b ). Similar to the first experiment, subjects would not be able to prepare a motor response until action cue onset, even though the behaviourally relevant visual stimulus was evident right from RDK onset. As in Experiment 1, discrimination performance increased for higher motion coherences (mean accuracy for 5/15/30/70% coherence: 0.35/0.55/0.80/0.91), as did decision confidence (mean certainty index for 5/15/30/70% coherence: 0.40/0.50/0.73/0.92; Fig. 1f ). RTs varied with stimulus properties: responses were significantly faster for correct motion discrimination (mean correct=4.275±0.282 s, mean incorrect=4.399±0.289 s; t -test: P =0.001). Subjects were faster to respond to higher coherence levels with a significant difference of highest and lowest coherence (mean for 70% coherence=4.245±0.281 s, mean 5%=4.379±0.296 s; t -test: P =0.003). RTs were faster with higher choice certainty, with significant differences between highest and lowest confidence levels (mean for certainty 3 =4.210±0.261 s, mean 0 =4.426±0.266 s; t -test: P =0.001). 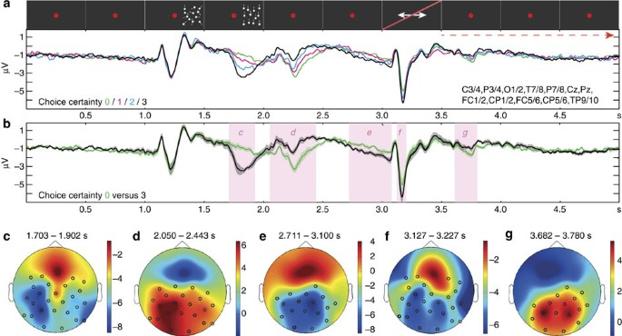Figure 7: Differences between confidence ratings in Experiment 2. (a) Symbolic representation of the visual stimulus along the stimulus-locked grand-average ERP responses. Different colours represent ERPs for the four different confidence ratings, on a scale of 0–3 (from0being ‘I guessed’, to3‘I was sure’). (b) Stimulus-locked grand-average ERP responses to highest and lowest confidence ratings differed in five time intervals (indicated by pink areas). (c–g) Headplots of the nonparametric cluster-randomization approach (two-tailedt-test, corrected for multiple comparisons at a cluster-level,P<0.050) map the scalp distribution of statistical differences of ‘I was sure’ versus ‘I guessed’ ratings. Heat colours of the maps represent thet-values of the statistical comparisons (colour bar indicatest-values, relative scaling is specific to each topoplot) and the black circles represent electrodes that contribute to the significant cluster. (c) Negative cluster from 1.703 to 1.902 s (P=0.003). (d) Positive cluster from 2.050 to 2.443 s (P<0.001). (e) Negative cluster from 2.711 to 3.100 s (P=0.003). (f) Negative cluster from 3.127 to 3.227 s (P=0.014). (g) Positive cluster from 3.682 to 3.780 s (P=0.039). ERP responses are averages over all electrodes of cluster (d) and are plotted with s.e. values of the mean (shaded areas). Figure 7a overlays the grand-average event-related potentials (ERPs) of the subjects’ four certainty levels time-locked to the onset of the trials. With the omission of the selective attention instruction of Experiment 1, ERPs changed considerably. While prestimulus RDK onset at 1.0 s and the appearance of the action cue at 3.0 s evoked classical N100 and P200 effects (see for example, Experiment 1), we observed five pronounced dissociations of brain electrical activity with different polarities and localizations. In a statistical comparison of lowest and highest certainty trials ( Fig. 7b ), these dissociations were expressed by three significant negative clusters over parieto-occipital electrodes that were present from 1.703 to 1.902 s ( P =0.003), 2.711 to 3.100 s ( P =0.003), and 3.127 to 3.227 s ( P =0.014); as well as by two positive clusters from 2.050 to 2.443 s ( P <0.001; electrodes plotted in ERPs) and 3.682 to 3.780 s ( P =0.039). Consistent with the controls in Experiment 1, in the second experiment we inspected the contrast of lowest and highest certainty trials for the influence of the presented motion coherence. 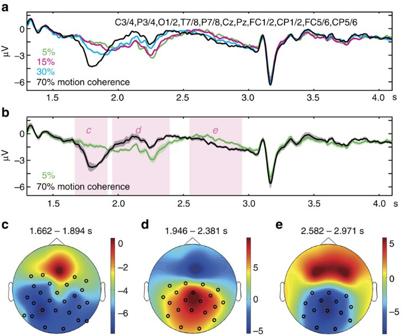Figure 8: Differences between presented motion coherence levels in Experiment 2. (a) Stimulus-locked grand-average coherence ERP responses. Different colours represent ERPs for the four different levels of motion coherence (5, 15, 30 and 70%) presented in the experiment. (b) Stimulus-locked grand-average ERP responses to the highest and the lowest coherence level differed in three time intervals (indicated by pink areas). (c–e) Headplots of the nonparametric cluster-randomization approach (two-tailedt-test, corrected for multiple comparisons at a cluster-level,P<0.050) map the scalp distribution of statistical differences of 70 versus 5% motion coherence. Same conventions as inFig. 2, colour bar indicatest-values, relative scaling is specific to each topoplot. (c) Negative cluster from 1.662 to 1.894 s (P=0.007). (d) Positive cluster from 1.946 to 2.381 s (P<0.001). (e) Negative cluster from 2.582 to 2.971 s (P=0.005). ERP responses are averages over electrodes of cluster (d) and are plotted with s.e. values of the mean (shaded areas) inb. Figure 8a side-by-side displays the ERPs for the four motion coherence levels—5, 15, 30 and 70%—presented in Experiment 2 and the results of the cluster statistics. Randomization tests identified larger negative deflections over parieto-occipital electrodes for 70% motion coherence as compared with 5% coherence from 1.662 to 1.894 s ( P =0.007) and from 2.582 to 2.971 s ( P =0.005); as well as a larger positive deflection for this contrast from 1.946 to 2.381 s ( P <0.001; electrodes plotted in ERPs). Higher motion coherence in more certain responses—12.88% for certainty rating 0 , 17.73% for 1 , 33.83% for 2 , 50.59% for 3 —could account for the early certainty ERP differences, but could not for the ERP dissociations after the action cue (see for example, Figs 7b and 8b ). Again, that motivated further controls for covariance of certainty with further stimulus properties or subjects’ performance. We first inspected ERPs of highest versus lowest confidence ratings for correct answers ( Fig. 9a ). In a next step, we examined the certainty contrast for a combined grand average of single subjects’ 15 and 30% motion coherence averages as there were not enough high certainty trials for the 15% coherence level and not enough low certainty trials for the 30% coherence level to generate separate averages that were adequate for cluster statistics ( Fig. 9b ). While the significant ERP dissociations are marked for all pools of trials, to avoid redundancy the topography of the significant clusters is just detailed for the most rigorous of the controls that is the intersection of these two pools of trials ( Fig. 9c ). In contrast to Experiment 1, the early dissociation during stimulus presentation proved significant for all three pools of trials, most notably for the two coherence controls in Fig. 9b,c , as well. This certainty correlate was represented by a significant negative cluster from 1.803 to 1.850 s ( P =0.020). During the interval leading from stimulus offset to the action cue ERP differences were expressed by two significant positive clusters from 2.246 to 2.292 s ( P =0.009) and from 2.300 to 2.355 ( P =0.009), respectively, as well as two significant negative clusters from 2.892 to 2.954 s ( P =0.019) and from 3.148 to 3.203 s ( P =0.034). All five ERP activations indicative of choice certainty, thus, were not confounded by the presented motion coherence. Figure 7: Differences between confidence ratings in Experiment 2. ( a ) Symbolic representation of the visual stimulus along the stimulus-locked grand-average ERP responses. Different colours represent ERPs for the four different confidence ratings, on a scale of 0–3 (from 0 being ‘I guessed’, to 3 ‘I was sure’). ( b ) Stimulus-locked grand-average ERP responses to highest and lowest confidence ratings differed in five time intervals (indicated by pink areas). ( c – g ) Headplots of the nonparametric cluster-randomization approach (two-tailed t -test, corrected for multiple comparisons at a cluster-level, P <0.050) map the scalp distribution of statistical differences of ‘I was sure’ versus ‘I guessed’ ratings. Heat colours of the maps represent the t -values of the statistical comparisons (colour bar indicates t -values, relative scaling is specific to each topoplot) and the black circles represent electrodes that contribute to the significant cluster. ( c ) Negative cluster from 1.703 to 1.902 s ( P =0.003). ( d ) Positive cluster from 2.050 to 2.443 s ( P <0.001). ( e ) Negative cluster from 2.711 to 3.100 s ( P =0.003). ( f ) Negative cluster from 3.127 to 3.227 s ( P =0.014). ( g ) Positive cluster from 3.682 to 3.780 s ( P =0.039). ERP responses are averages over all electrodes of cluster ( d ) and are plotted with s.e. values of the mean (shaded areas). Full size image Figure 8: Differences between presented motion coherence levels in Experiment 2. ( a ) Stimulus-locked grand-average coherence ERP responses. Different colours represent ERPs for the four different levels of motion coherence (5, 15, 30 and 70%) presented in the experiment. ( b ) Stimulus-locked grand-average ERP responses to the highest and the lowest coherence level differed in three time intervals (indicated by pink areas). ( c – e ) Headplots of the nonparametric cluster-randomization approach (two-tailed t -test, corrected for multiple comparisons at a cluster-level, P <0.050) map the scalp distribution of statistical differences of 70 versus 5% motion coherence. Same conventions as in Fig. 2 , colour bar indicates t -values, relative scaling is specific to each topoplot. ( c ) Negative cluster from 1.662 to 1.894 s ( P =0.007). ( d ) Positive cluster from 1.946 to 2.381 s ( P <0.001). ( e ) Negative cluster from 2.582 to 2.971 s ( P =0.005). ERP responses are averages over electrodes of cluster ( d ) and are plotted with s.e. values of the mean (shaded areas) in b . 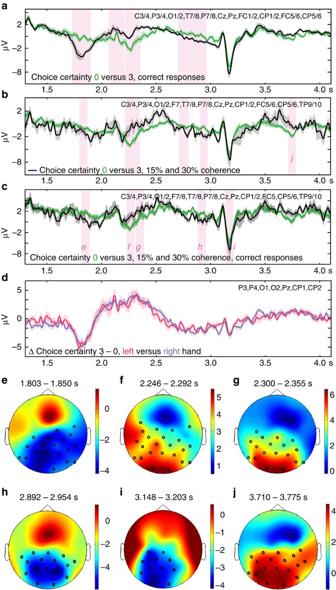Figure 9: Certainty correlates for Experiment 2. (a–c) Stimulus-locked grand-average ERP responses to highest versus lowest confidence ratings: (a) for correct responses only, (b) for an average of 15 and 30% motion coherence, (c) for correct responses in 15 and 30% motion coherence trials. Each of the three ERP contrasts (a–c) differed in rather similar time intervals (indicated by pink areas). Please note that with more restrictive selection criteria fromatocthe size of the respective pool of trials decreased considerably. (d) Stimulus-locked ERPs of certainty-specific activity (Δ choice certainty3−0) for left versus right hand responses. Cluster statistics inddid not reveal a significant dissociation of Δ choice certainty ERPs for left versus right hand responses. (e–j) Headplots of the nonparametric cluster-randomization approach (two-tailedt-test, corrected for multiple comparisons at a cluster-level,P<0.050) map the scalp distribution of statistical differences of ‘I was sure’ versus ‘I guessed’ ratings. Heat colours of the maps represent thet-values of the statistical comparisons (colour bar indicatest-values, relative scaling is specific to each topoplot) and the black circles represent electrodes that contribute to the significant cluster. While the significant ERP dissociations are marked for all three pools of trials, to avoid redundancy the topography of the significant clusters is just detailed for the most rigorous of the controls that is the intersection of these two pools of trials (c). (e) Negative cluster from 1.803 to 1.850 s (P=0.020). (f) Positive cluster from 2.246 to 2.292 s (P=0.009). (g) Positive cluster from 2.300 to 2.355 (P=0.009). (h) Negative cluster from 2.892 to 2.954 s (P=0.019). (i) Negative cluster from 3.148 to 3.203 s (P=0.034). (j) Positive cluster from 3.710 to 3.775 s (P=0.012). ERP responses are averages over all electrodes that were part of the respective significant cluster and are plotted with s.e. values of the mean (shaded areas). Full size image Figure 9: Certainty correlates for Experiment 2. ( a – c ) Stimulus-locked grand-average ERP responses to highest versus lowest confidence ratings: ( a ) for correct responses only, ( b ) for an average of 15 and 30% motion coherence, ( c ) for correct responses in 15 and 30% motion coherence trials. Each of the three ERP contrasts ( a – c ) differed in rather similar time intervals (indicated by pink areas). Please note that with more restrictive selection criteria from a to c the size of the respective pool of trials decreased considerably. ( d ) Stimulus-locked ERPs of certainty-specific activity (Δ choice certainty 3 − 0 ) for left versus right hand responses. Cluster statistics in d did not reveal a significant dissociation of Δ choice certainty ERPs for left versus right hand responses. ( e – j ) Headplots of the nonparametric cluster-randomization approach (two-tailed t -test, corrected for multiple comparisons at a cluster-level, P <0.050) map the scalp distribution of statistical differences of ‘I was sure’ versus ‘I guessed’ ratings. Heat colours of the maps represent the t -values of the statistical comparisons (colour bar indicates t -values, relative scaling is specific to each topoplot) and the black circles represent electrodes that contribute to the significant cluster. While the significant ERP dissociations are marked for all three pools of trials, to avoid redundancy the topography of the significant clusters is just detailed for the most rigorous of the controls that is the intersection of these two pools of trials ( c ). ( e ) Negative cluster from 1.803 to 1.850 s ( P =0.020). ( f ) Positive cluster from 2.246 to 2.292 s ( P =0.009). ( g ) Positive cluster from 2.300 to 2.355 ( P =0.009). ( h ) Negative cluster from 2.892 to 2.954 s ( P =0.019). ( i ) Negative cluster from 3.148 to 3.203 s ( P =0.034). ( j ) Positive cluster from 3.710 to 3.775 s ( P =0.012). ERP responses are averages over all electrodes that were part of the respective significant cluster and are plotted with s.e. values of the mean (shaded areas). Full size image The late, significant dissociation seen in the pooled data above ( Fig. 7g ) was detected for the second control only ( Fig. 9j ) but missed significance in the other two controls. It was expressed by a significant positive cluster of parieto-occipital electrodes from 3.710 to 3.775 s ( P =0.012). Again, we found a significant difference between response times for highest and lowest certainty (mean RT for highest certainty 4.184 s versus lowest 4.393 s; t -test: P =0.002). This difference was also significant when left hand (4.237 s versus 4.441 s; t -test: P =0.001) and right hand responses (4.187 s versus 4.411 s; t -test: P <0.001) were analysed separately. A statistical comparison of confidence-specific ERP activity (Δ certainty 3 − 0 ) did not show a significant difference between right and left hand responses ( Fig. 9d ). This control demonstrated that correlates of choice certainty did not depend on the motor effector. The present study was performed to systematically manipulate the level of selective attention and motor effectors, and relate both to objective performance and subjective confidence as well as to electrophysiological correlates of visual perceptual certainty. Consistent with previous studies [12] , [16] decision confidence correlated with different experimental variables, that is, sensory evidence, selective attention and motor response times as expected. We performed strict controls to establish specific correlates of choice certainty not confounded by these covariances. Indeed, ERP variations with motion coherence and spatial cueing could have been mistaken for primary representations of decision confidence. Visual-evoked ERP activity started to differ significantly between the four levels of motion coherence as early as ~170 ms after stimulus onset ( Fig. 5f ). The cortical activity that gave rise to this effect and linearly increased with motion coherence is likely to reflect compound activitiy of large parts of motion sensitive visual cortex including, among others, areas MT/MST, V3A, and also parietal cortex (see for example, Figs 2 , 4 and 5 ). Neurons in area MT have been shown to linearly increase firing rate with motion coherence in various single-cell recording studies [17] , [18] and the strength of visual motion is reflected in human area MT + activity in fMRI [19] , [20] , [21] , MEG [13] and EEG data [22] . Interestingly, the evoked activity following invalid postcues in our Experiment 1 also varied with attributes of the visual stimulus, that is, motion coherence ( Fig. 5g ). Its spatial distribution very much resembled the early visual-evoked potential reflecting motion strength ( Fig. 5f ). This suggests that parts of the motion-sensitive cortex were reactivated following invalid postcues, even though the visual motion stimulus was not repeated. In other words, invalid cueing apparently induced a retrieval of motion information from working memory finally resulting in the perceptual decision [23] . A classic P300 potential following the less frequent invalid cues varied with motion coherence, as well ( Fig. 5h ). While the exact mechanisms underlying perceptual decisions in invalid cue trials were not within the scope of our experiments, the statistical comparisons confined to a single coherence levels or attention condition allowed us to decide on whether a possible ERP correlate of choice certainty was secondary to stimulus properties or attentional states. Following that approach, our findings revealed a sequence of ERP responses indicative of subjective confidence. The first certainty correlate was observed during the presentation of the test stimulus. Capitalizing on the EEG’s high temporal precision, our data let us determine when perceptual confidence forms in the visual pathway. In Experiment 2, certainty-specific ERP activity, independent of the presented motion coherence, followed stimulus onset by ~300 ms ( Fig. 9c ). Correlates of perceived confidence thus emerged ~130 ms later than representations of motion coherence that followed stimulus onset by ~170 ms (see for example, Fig. 9c versus Figs 5c,d and 8b). Perceptual decision confidence thus evolved nearly in parallel with representations of stimulus properties. The distribution of this early certainty-specific ERP activity was very similar to the cortical topography of the sensory evidence suggesting a shared neurophysiological substrate. Subsequent distinct correlates of perceived confidence were identified during the 1,000 ms leading to the action cue ( Fig. 9f–h ). These certainty correlates in the EEG signal during the fixation period between RDK offset and action cue onset were enhanced over parieto-occipital electrodes, as well, and changed polarity once during the 1,000 ms interval. In contrast to Experiment 1, Fig. 7b displays certainty-specific ERP activity during stimulus presentation in the second experiment, and later anew during the following fixation, that is not confounded by sensory evidence or objective discrimination performance (see for example Fig. 9a–c ). Moreover, by keeping the signal-to-noise ratio constant ( Figs 6b and 9b ) we illustrated that the certainty correlates were not confounded by a task-difficulty component or noise-induced modulation of sensory processing demands [24] . Both experiments, however, revealed an electrophysiological correlate of decision confidence during the time interval leading from the postcue in Experiment 1 or action cue in Experiment 2, respectively, to the motor response. This correlate was not confounded by stimulus or response characteristics either (see for example Figs 6a–c and 9b ). Why did the two perceptual tasks differ with respect to the certainty-specific ERP activity detected in the course of the experiment? We started our discussion with Experiment 2 that featured a slightly simpler experimental design. Most notably, it did not include attention cueing, but randomly varied the instruction as to which effector (right or left hand) to use for the motor response. In Experiment 1, ERPs time-locked to the visual stimulus showed significant differences in brain electrical activity with decision confidence for pooled data ( Fig. 2 ) and separate cueing conditions alike ( Fig. 4 ). But in contrast to Experiment 2, controls for the influence of presented motion coherence demonstrated that it was more parsimonious to assume that the correlation of this ERP component with certainty was due to its covariance with presented motion coherence ( Fig. 6 ). Since mean motion coherence was higher in more certain responses, ERP differences seen in Experiment 1 for the different certainty levels during test stimulus presentation thus could be explained most parsimoniously by electrophysiological correlates of visual motion processing, that is, by differences in sensory evidence. While this was also true for the early part of the certainty correlate during stimulus presentation in Experiment 2, we observed distinct correlates of perceived confidence emerging about ~130 ms later than representations of motion coherence that followed stimulus onset by ~170 ms (see for example, Fig. 9c ). The subsequent certainty-specific activations during the 1,000 ms after stimulus offset were not present at all in Experiment 1. As the course of the two experiments is similar except for attention cueing, we propose that choice certainty does not evolve unless or until decision variables are unambiguous. Although stimuli were cued validly in 80% of the trials in Experiment 1, obviously subjects would not attribute certainty to one of the two random dot stimuli until the instructional postcue clearly indicated which of the two was relevant to behaviour. Confidence thus appears to form only if the target of interest is unambiguous. This observation suggests that perceptual confidence—like the decision process itself—is unitary and assigned to one specific aspect of the visual world but not shared across different items. Then again, this perspective implies that subjects were not able to completely ignore the distractor stimulus, even though their behavioural data show that they followed the attention instruction. Apparently subjects to some extent divided their spatial attention—a mode of behaviour controversially debated in the previous literature [25] , [26] —or shifted spatial attention in time. The latest of the certainty correlates in the course of the first experiment appeared in valid cue trials only (see for example, Fig. 4c versus Fig. 4d). The onset of the significant confidence-specific cluster ( Fig. 6d–f ) preceded the motor response by about 300 ms relating to the mean response time of highest and lowest confidence ratings. In that all our subjects indicated perceived motion direction by finger movements of their right hand in Experiment 1, this activity’s focus over left parietal cortex motivated further controls for the potential confounder of motor contributions to the responses. As mean response times for highest and lowest certainty ratings differed significantly, we aligned the ERPs to the response (first button press) to control for the potential confounder of motor contributions to the responses ( Fig. 6g ). ERPs did not show relevant certainty-specific activity time-locked to the response within the 400 ms preceding the button press. To comprehensively elucidate the possible role of choice certainty in motion preparation, Experiment 2 did not include attention cueing, but randomly varied the instruction as to which motor effector to use for the response. The late ERP response observed for valid trials in Experiment 1 was replicated in the second experiment with very similar temporal and spatial characteristics ( Figs 7g and 9j ). The design of the second task made a comparison of the ERPs of right and left hand responses possible that did not show a significant difference in confidence-specific ERP activity (Δ certainty 3 − 0 ) between effectors. While timing and location of the late ERP dissociation with choice certainty suggested a correlation with premotor activity, the ERP difference evidently was neither locked to the motor response nor specific to the movement effector. Electrophysiological correlates of decision confidence preceded the motor response, but were neither essential for nor obligatorily linked to its emergence. Moreover, the absence of effector-specific ERP activity in this hemispheric contrast made the possiblity implausible that the certainty dissociation preceding the motor response represented movement execution itself. Both in Experiment 1 and 2 controls for the confounding factor motion coherence ( Figs 6b and 9b ) made it improbable that the late ERP dissociation represented more frontal contributions to working memory for visual motion observed in previous moving random-dot experiments [27] . Rather one may well ask whether electrophysiological or imaging findings are—at least for comparable discrimination tasks—confounded by correlates of subjective confidence in the perceptual decision. Earlier in this discussion we have established that decision confidence in Experiment 1 is not traceable before subjects finally commit to a hemifield stimulus or post-cue instruction, respectively, and attention therefore is no longer divided. For invalid cues in Experiment 1, there was no certainty-specific activity present, as all confidence correlates were confounded by the presented motion coherence ( Fig. 5d ). In this line of argument, the ERP dissociation with motion coherence following the post-cue instruction in invalid cue trials may represent the reactivation and concluding evaluation of stimulus-specific and certainty information after a ‘surprising’ turn of events requiring to start the perceptual decision again. To hypothesize further, the recall of stimulus characteristics in invalid cues may not have been sufficient for detectable confidence correlates to develop. Without selective attention cueing, in Experiment 2 perceptual stimulus information entered a fundamentally different stream of cortical processing right after RDK presentation that did not require later reactivation. While the evaluative processes in perceptual decision making doubtless culminate in the completion of the decision, it might be speculated that peri-decisional processes like decision confidence determine how chosen decisions are maintained, protected from competing alternatives and enacted [28] . Choice certainty in this model is an aspect of metacognition that represents the investment of significant resources in the process by which decisions are reached. It motivates subsequent pursuit or effort investment and benefits eventual realization as a high confidence decision is more likely to be enacted than one fraught with uncertainty [29] . We hypothesize that as a consequence choice certainty correlates are perpetuated in preparation of a motor response. In conclusion, our findings reveal electrophysiological correlates of subjective experience. A succession of ERP correlates each reflecting perceptual decision confidence is independent of objective performance and overt behaviour. Choice certainty evolves in parallel with representations of the visual stimulus and emerges ~130 ms later than representations of motion coherence. The certainty-specific ERP activity topographically resembles representations of the sensory evidence suggesting a similar neurophysiological substrate. Representations of choice certainty over parieto-occipital cortex are not detectable unless or until attention is no longer divided and persist beyond stimulus presentation. These distinct correlates are identified during the interval leading to the motor response, but are independent of movement execution and do not differentiate between motor effectors. A decision-theoretic framework that accounts for choice certainty may help to improve our understanding of sensory-guided behaviour. Beyond that, of course, human decision making extends to abstract decisions about propositions independent of what, if anything, will be done as a consequence. With separate streams of partial evidence flowing continuously to the integrators of subsequent decisions [30] , it seems likely that the principles and mechanisms of simple perceptual decisions also support complex cognitive functions and decision confidence is represented at this level of integration. Subjects Thirteen subjects were tested in Experiment 1, data from three subjects were discarded due to excessive eye blinking or muscle artefacts, leaving one left-handed and nine right-handed participants (three females; mean age=23.5 years) in the final analysis. Twelve more subjects participated in Experiment 2, data from two subjects were discarded since the highest certainty level (see below) was used too infrequently (<2% of trials), leaving ten right-handed participants (five females; mean age=23.5 years). All subjects had normal or corrected-to-normal visual acuity and reported to be free of neurological or psychiatric impairment. Written informed consent was obtained from all subjects according to the Declaration of Helsinki and the guidelines of the local ethics committee of the faculty of medicine of the University of Tübingen, which approved the procedures. Design and procedures To explore electrophysiological correlates of objective and subjective performance with and without selective attention, we designed two visual motion perception experiments using RDKs. In Experiment 1, a spatial attention precue-postcue experiment, subjects were instructed to stringently follow an attention cue preceding the stimulus. Participants always had to discriminate the global direction of one of two motion stimuli presented simultaneously differing in location. They would not respond before a postcue indicated which of the two stimuli they actually had to evaluate. Both a decision and the confidence in it was given trial by trial, all subjects followed the instructions as illustrated by changes of objective performance with attention. EEG was recorded continuously during the course of the experiment. The visual stimulus consisted of six periods, each lasting 500 ms except for the second fixation period, which lasted 1,000 ms (see Fig. 1a ). After a first fixation period (central fixation dot, red, diameter 2 arcmin; 500 ms) a central arrow (dimensions: 3°x1°, white, luminance 384 cd m −2 ; 500 ms) instructed subjects to covertly shift attention either to the left or right hemifield. This attention cue was followed by two RDKs, each of which covered a square of 9° × 9° and was centred 13° right and left, respectively, of the fixation point. Each RDK consisted of 475 white squares (side length=0.8 arcmin, lifetime=500 ms, dot density ~6 dots deg −2 , luminance 384 cd m −2 ) on a black background (luminance 0.14 cd m −2 ), all moving incoherently, that is, in all possible directions with a resolution of 1°, at a common speed of 6 deg s −1 . After the presentation of this first pair of RDKs (prestimulus; 500 ms), a second pair of RDKs, the test stimulus, started and was presented for 500 ms [13] , [14] . The properties of the test stimulus were identical to those described for the prestimulus except that a certain percentage of the dot elements moved coherently in the same direction (either up, right, down or left). The percentage of coherently moving dots in an individual trial was chosen equally and randomly from four predefined steps (10, 20, 30 or 40% of all dots). Motion coherence was always identical for the two RDKs in a given trial, global motion direction could be the same or different as randomly chosen by the computer. After a subsequent second fixation period (1,000 ms), a second arrow presented for 500 ms indicated for which of the two RDKs subjects had to report the direction of coherent motion (four-alternative forced choice). Valid cueing—as defined by congruent orientation of the precue and the postcue—was applied in 80% of trials. Subjects reported their post-decision certainty by pressing one of four buttons used to signal the perceived motion direction right before. Uniformly, subjects were asked to rate how confident they were in their decision on a scale of 0–3 ( 0 being ‘I guessed’, 3 ‘I was sure’, 1 and 2 equally spaced steps of the continuum in between), distributing their responses over the available scaling. Both responses were given starting at 3.5 s using the right hand only and had to be completed within 7 s for a trial to be counted, after the second key press a new trial would start automatically. An initial practice run of 50–70 trials familiarized the subjects with the procedure and stabilized discrimination thresholds; these trials were not used for further analysis. Each subject completed about 1,300 trials and was offered several breaks. Subjects viewed all stimuli binocularly from a distance of 55 cm on a 19” TFT-display (native resolution 1,280 × 1,024 pixels) driven by a Linux computer running the open source nrec visual stimulation, data acquisition and experiment control software package ( http://nrec.neurologie.uni-tuebingen.de , created by F. Bunjes, J. Gukelberger et al .) at a refresh rate of 60 Hz in a dark, quiet room. In Experiment 2, participants were guided to discriminate the global direction of one motion stimulus presented either right or left of the fixation point. Other than in Experiment 1, there was neither an instruction to shift attention nor a second RDK presented simultaneously with the test stimulus. Subjects would not respond before an arrow pointing left or right indicated which hand they had to respond with, respectively. Both the decision and the confidence in it were given trial by trial by using the response device with the instructed hand. The visual stimulus consisted of five periods, each lasting 500 ms except for the two fixation periods that lasted 1,000 ms (see Fig. 1b ). Stimulus and response specifications were otherwise identical to Experiment 1 except for the test stimulus being presented randomly in the right or left visual hemifield, the absence of an attentional cue and the four predefined coherence levels being 5, 15, 30 and 70% of all dots. On the basis of the preliminary perceptual thresholds of Experiment 1, the coherence levels in the second experiment were chosen differently to better balance the subjects’ certainty ratings for the statistical analysis. Both responses were given starting at 3.5 s and had to be completed within 7 s for a trial to be counted. After an initial practice run of 50–70 trials, each subject completed about 800 trials and was offered at least two breaks. EEG was recorded continuously during the course of the experiment. Eye movement recordings During the entire course of a single trial, subjects would fixate the central fixation dot while eye movements were monitored using a custom-built video system taking the pupil’s centre as measure of eye position. Recordings were recorded and stored at a sampling rate of 50 Hz and quality of fixation was analysed offline. In particular, deviations from the fixation point (eye position) were examined for the period of test stimulus presentation. All subjects maintained stable fixation as indicated by a mean horizontal (h) and vertical (v) eye positions close to 0° and small s.d. values: h:0.95°±2.52°, v-0.41°±1.84° in Experiment 1 and h:0.14°±3.01°, v-0.11°±3.11° in Experiment 2. Electrophysiological recordings EEG was recorded at 29 scalp sites (Fp1, Fp2, F3, F4, C3, C4, P3, P4, O1, O2, F7, F8, T7, T8, P7, P8, Fz, Cz, Pz, FC1, FC2, CP1, CP2, FC5, FC6, CP5, CP6, TP9 and TP10) versus the additional FCz electrode using an electrode cap equipped with Ag/AgCl electrodes (Easycap, Herrsching, Germany). The electro-oculogram (EOG) was monitored using an additional electrode placed below the lateral canthus of the right eye. The impedance of the electrodes was kept below 10 kΩ, EEG and EOG signals were amplified using a 32-channel BrainAmp EEG amplifier (Brainproducts, Munich, Germany). All signals were continuously sampled at 1,000 Hz and filtered using a band-pass filter from 0.53 Hz to 35 Hz. Data analysis Data analyses were performed with custom-made software based on MATLAB (Mathworks, Natick, MA) and the Fieldtrip toolbox [31] . EEG data were corrected for eye movement artefacts using independent component analysis via CORRMAP [32] within EEGLAB [33] in Experiment 1 and using Fieldtrip ICA correction in Experiment 2. All trials then were visually inspected and trials with remaining artefacts were excluded from analysis. To compare accuracy and certainty data psychophysically, a certainty index was defined that reflects the stochastics of the task and subjects’ instructions. Confidence 0 /left button was coded 0.25; 1 /up button 0.50; 2 /right button 0.75; 3 /down button 1. Subjects’ mean accuracy ( Fig. 1c ) and certainty of all coherence levels for valid and invalid cues ( Fig. 1d ) were z-transformed to a common mean (0) and s.d. (1) in Experiment 1. Standardized accuracy measures for valid and invalid cueing were subjected to paired t -tests, as were standardized certainty measures. Paired differences of valid and invalid accuracy measures (Δ z-values) were compared with corresponding certainty deltas in a paired t -test to examine the effects of attention on both objective and subjective performance ( Fig. 1e ). All response times refer to the beginning of the trial. ERPs were calculated relative to the onset of the trials with the first fixation period by averaging for each condition and subject separately. To test for significant differences between respective conditions, a cluster-randomization procedure [34] was applied that effectively controls the type I error rate in multiple comparisons by clustering neighbouring (electrode-time) pairs that differ significantly between conditions. First, two-sided t -tests were performed and thresholded (α=0.050) for the difference between two conditions for individual electrode-time pairs. Then, significant electrode-time pairs were clustered by identifying pairs showing the same direction of effect. For each cluster, a cluster-level statistic was calculated by taking the sum of all the individual t -statistics within that cluster. The Type I error rate was controlled by evaluating the cluster-level statistics under a randomization null distribution of the maximum cluster-level statistic. This randomization null distribution was obtained by randomizing the data between conditions across participants in 10,000 randomizations. Finally, the actually observed cluster-level statistic was compared with the randomization null distribution. The P -value was estimated as the proportion of the randomization null distribution in which the maximum cluster-level test statistics exceeded the observed maximum cluster-level test statistic. Clusters that had a P -value below 0.050 were considered significant. How to cite this article: Zizlsperger, L. et al . Cortical representations of confidence in a visual perceptual decision. Nat. Commun. 5:3940 doi: 10.1038/ncomms4940 (2014).